Role of Rab11 in planar cell polarity and apical constriction during vertebrate neural tube closure Epithelial folding is a critical process underlying many morphogenetic events including vertebrate neural tube closure, however, its spatial regulation is largely unknown. Here we show that during neural tube formation Rab11-positive recycling endosomes acquire bilaterally symmetric distribution in the Xenopus neural plate, being enriched at medial apical cell junctions. This mediolateral polarization was under the control of planar cell polarity (PCP) signalling, was necessary for neural plate folding and was accompanied by the polarization of the exocyst component Sec15. Our further experiments demonstrate that similar PCP-dependent polarization of Rab11 is essential for ectopic apical constriction driven by the actin-binding protein Shroom and during embryonic wound repair. We propose that anisotropic membrane trafficking has key roles in diverse morphogenetic behaviours of individual cells and propagates in a tissue by a common mechanism that involves PCP. Epithelial tissue folding is a universal mechanism for germ layer rearrangements at gastrulation, neural tube closure and organogenesis. During vertebrate neurulation, dorsal ectoderm forms the neural plate that bends to generate the neural groove [1] , [2] , [3] . At a later stage, the bilateral neural folds fuse at the midline into the neural tube. Actomyosin contractility and cell junction remodelling are believed to be major driving forces for epithelial folding in Drosophila embryos [2] , [3] , [4] , [5] , apical constriction in C. elegans endoderm progenitors [6] and during vertebrate neural tube closure [7] , [8] , [9] , [10] . In addition, mutations in genes encoding core planar cell polarity (PCP) proteins Frizzled, Dishevelled, Vangl2/Strabismus, Flamingo/Celsr and Prickle reveal neural tube defects (reviewed by Bayly and Axelrod [11] , Zallen [11] and Wallingford et al. [13] ). Although PCP signalling has been linked to Rho signalling and actomyosin contractility in gastrulation and neurulation [9] , [14] , [15] , [16] , molecular mechanisms underlying neural tube defects in PCP mutants are still unknown. In Xenopus neural plate explants, deep layer cells display monopolar protrusive activity towards the midline [17] , yet molecular markers of this polarization have not been identified and whether this polarity relates to apical constriction that occurs at the hinge regions of the bending neural plate is unclear. As membrane trafficking has essential roles in diverse morphogenetic events, including cell intercalation [15] , epithelial polarization [18] , [19] and neural tube formation [20] , we examined potential functions for endocytic proteins that might be associated with morphological changes during Xenopus neural plate closure. We were especially interested in Rab11, a recycling endosome marker with roles in cell polarity and cell migration [21] , [22] , [23] , [24] , [25] . Our results reveal unique planar polarization of Rab11 in the neural plate, which is regulated by PCP signalling and which is essential for neural tube formation. Planar polarization of Rab11 in the neural plate Immunostaining of sectioned early neurula embryos at stages 14–15 revealed striking polarization of Rab11 in the plane of the neuroepithelium ( Fig. 1a–c , Supplementary Fig. 1a–d ). Even before neural plate folding became morphologically apparent, Rab11 became localized to one apical corner of neuroepithelial cells that is closer to the dorsal midline, thereby establishing mirror-image planar polarity in the early neural plate. The bilateral staining progressively changed towards apical midline staining at the neural fold stages ( Fig. 1a,b , Supplementary Fig. 1a,b ). Other apical or basolateral markers, such as atypical PKC, ZO1 and β-catenin, did not reveal similar polarization ( Fig. 1c–e ). The observed pattern was often detected as comet-shape cytoplasmic staining directed towards a cell junction (marked by ZO1, Fig. 1d ). To independently confirm that Rab11 is indeed unilaterally polarized in individual cells, we examined early embryos injected with RNA-encoding Rab11-green fluorescent protein (GFP; Fig. 1f ). Mosaically expressed exogenous Rab11-GFP was similarly distributed in a gradient with the highest concentration at the medial apical corner of the cell ( Fig. 1f ). Lack of staining in the neighboring cells, which did not receive Rab11-GFP RNA, allowed us to unequivocally define the position of Rab11-GFP relative to the cell border. En face views of the neural plate immunostained for both endogenous and exogenous Rab11 confirmed the polarization of Rab11 in the plane of the tissue, in a manner reminiscent of the distribution of PCP proteins in Drosophila epithelia [11] ( Fig. 1g–i ). Interestingly, Diversin, a vertebrate homologue of the fly PCP protein Diego, revealed a similar polarization ( Fig. 1i,i′ ), providing insight into the role of PCP proteins in neural tube closure. These findings suggest that anisotropic Rab11-dependent recycling is an early event in neural tube closure. 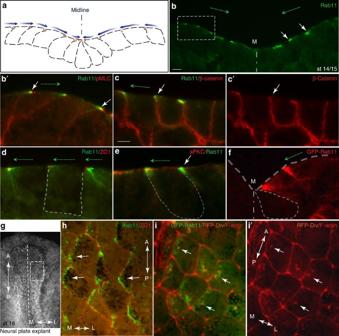Figure 1: Rab11 distribution reveals planar polarity along the mediolateral axis of theXenopusneural plate. (a,b) Scheme (a) and a representative transverse cryosection (b) of the neural plate stained with anti-Rab11 monoclonal antibodies at stage 14/15. (b′) Higher magnification is shown for image within the white square inb. Costaining for phosphorylated myosin II light chain (pMLC,b′) reveals cell boundaries. (c–e) Embryo sections were co-stained with Rab11 and β-catenin (c,c′), ZO-1 (d) and aPKC (e) antibodies at higher magnification. (f) Polarized localization of exogenous Rab11. Four-cell embryos were injected with 100 pg of green fluorescent protein (GFP)-Rab11 RNA and stained with anti-GFP antibodies at midneurula stages (st 16). (b–f) White arrows point to polarized Rab11 distribution. Dashed green arrows and blue arrows ina, directed towards the midline (M) indicate cell and tissue polarity. Neural plate and individual cell boundaries are shown by broken lines. (g–i)En faceview of the neural plate with polarized Rab11 and Diversin (white arrows). (g) Dorsal view of a neural plate explant (stage 16) with white rectangle indicating approximate location of images inhandi. A, anterior; L, lateral; M, medial; P, posterior. (h) Endogenous Rab11 is medially enriched along the mediolateral (ML) axis. (i,i′) Both exogenous GFP-Rab11 (green vesicles) and Diversin-RFP (i′, cytoplasmic red staining) show medial polarization along the ML axis (white arrows) and partly co-localize. Antibody specificity is indicated at the upper right corner of each panel. The anteroposterior (AP) axis is indicated. Scale bar inbandc(also refers to (d–f) is 10 μm. Figure 1: Rab11 distribution reveals planar polarity along the mediolateral axis of the Xenopus neural plate. ( a , b ) Scheme ( a ) and a representative transverse cryosection ( b ) of the neural plate stained with anti-Rab11 monoclonal antibodies at stage 14/15. ( b′ ) Higher magnification is shown for image within the white square in b . Costaining for phosphorylated myosin II light chain (pMLC, b ′) reveals cell boundaries. ( c – e ) Embryo sections were co-stained with Rab11 and β-catenin ( c , c ′), ZO-1 ( d ) and aPKC ( e ) antibodies at higher magnification. ( f ) Polarized localization of exogenous Rab11. Four-cell embryos were injected with 100 pg of green fluorescent protein (GFP)-Rab11 RNA and stained with anti-GFP antibodies at midneurula stages (st 16). ( b – f ) White arrows point to polarized Rab11 distribution. Dashed green arrows and blue arrows in a , directed towards the midline (M) indicate cell and tissue polarity. Neural plate and individual cell boundaries are shown by broken lines. ( g – i ) En face view of the neural plate with polarized Rab11 and Diversin (white arrows). ( g ) Dorsal view of a neural plate explant (stage 16) with white rectangle indicating approximate location of images in h and i . A, anterior; L, lateral; M, medial; P, posterior. ( h ) Endogenous Rab11 is medially enriched along the mediolateral (ML) axis. ( i , i ′) Both exogenous GFP-Rab11 (green vesicles) and Diversin-RFP ( i ′, cytoplasmic red staining) show medial polarization along the ML axis (white arrows) and partly co-localize. Antibody specificity is indicated at the upper right corner of each panel. The anteroposterior (AP) axis is indicated. Scale bar in b and c (also refers to ( d – f ) is 10 μm. Full size image Rab11 is required for Myosin activation and neural folding To test whether Rab11-mediated membrane trafficking is required for neural plate folding, we studied the phenotype of embryos microinjected with RNA-encoding Rab11S25N, a dominant negative construct [23] , which is distributed throughout the cytoplasm ( Supplementary Fig. 1e,f ). In the majority of injected embryos (85%, n =53), the neural plate remained open at the injected side, yet this defect was rescued by wild-type Rab11 RNA ( Fig. 2a,b ). Similar results have been obtained using a specific morpholino antisense oligonucleotide (MO; Fig. 2c,d ), which effectively depletes Rab11 in Xenopus embryos [23] . The accumulation of phosphorylated myosin II light chain (pMLC), a key RhoA-dependent regulatory process in neural tube closure [7] , [8] , [9] , [10] , failed to occur ( Fig. 3a–c ), complementing changes in neural fold and individual cell morphology ( Fig. 2e,f ; Supplementary Fig. 2a,b ). This observation indicates that Rab11 is required for Myosin II activation in the neural plate. Despite these changes in the contractile machinery, the apical–basal polarity markers aPKC and ZO1 were not affected ( Fig. 3d,e ). Together, our observations show that Rab11 is not just a marker for neuroepithelial progenitor polarity, but an essential modulator of neural tube closure. Lack of changes in the neural tissue markers Sox3 ( Figs 2g and 3f ) , Nrp1 and Rx1 ( Supplementary Fig. 2c,d ) indicates that Rab11 is not involved in cell fate determination during neural induction. To further understand how Rab11 regulates neural plate folding, we examined the localization of exocyst, a protein complex that targets post-Golgi secretory vesicles for subsequent membrane fusion during exocytosis [26] . We find that the Rab11-interacting exocyst component Sec15 (ref. 27 ) polarizes in the neural plate similar to Rab11 ( Fig. 2h ). This result suggests that Sec15 promotes neural tube closure by directing exocytosis near the medial surface of each cell. 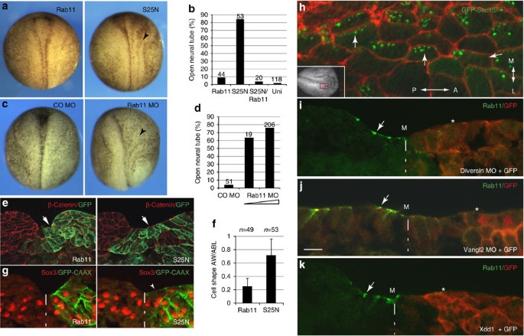Figure 2: Rab11 involvement in neural tube closure. (a–g) Four-cell embryos were injected unilaterally with Rab11 RNAs (1 ng) or morpholino antisense oligonucleotides (MOs; 20 ng) as indicated. Neural fold and cell morphology were assessed in whole embryos (a–d, dorsal view, anterior is at the top) and in cryosections (e–g). Rab11S25N and Rab11 MO, but not wild-type Rab11 or control MO, inhibit neural tube closure. Arrows point to neural folding defects. (b,d) Quantification of data presented inaandc. (e) Sections confirm the effect of Rab11S25N on neural fold morphology. β-Catenin staining reveals cell boundaries. (f) Ratios of apical width to apicobasal length (AW/ABL) in the neural groove cells that are adjacent to midline and express Rab11 constructs (stages 16/17;n, number of examined cells). Means±s.d. are shown on the graph. Rab11-expressing cells are indistinguishable from uninjected control cells (data not shown). (g) Rab11 constructs do not affect the neural progenitor fate marker Sox3. (h) Medial polarization of GFP-Sec15 in the neural plate of stage 15 embryos. Top view, red rectangle in the inset indicates approximate image position. F-actin marks cell boundaries. (i–k) Rab11 polarization depends on planar cell polarity. Immunostaining for endogenous Rab11 in cross-sections of stage 15/16 embryos unilaterally injected with Diversin MO (20 ng,i), Vangl2 MO (20 ng,j) or Xdd1 RNA (1 ng,k). Arrows point to polarized Rab11 on the uninjected side, asterisks indicate lack of Rab11 polarity. Scale bar inj(also refers toi,k) is 20 μm. M, midline position. GFP-CAAX or GFP RNA (100 pg) served as lineage tracers as indicated. Each result was verified in three to six independent experiments. Figure 2: Rab11 involvement in neural tube closure. ( a – g ) Four-cell embryos were injected unilaterally with Rab11 RNAs (1 ng) or morpholino antisense oligonucleotides (MOs; 20 ng) as indicated. Neural fold and cell morphology were assessed in whole embryos ( a – d , dorsal view, anterior is at the top) and in cryosections ( e – g ). Rab11S25N and Rab11 MO, but not wild-type Rab11 or control MO, inhibit neural tube closure. Arrows point to neural folding defects. ( b , d ) Quantification of data presented in a and c . ( e ) Sections confirm the effect of Rab11S25N on neural fold morphology. β-Catenin staining reveals cell boundaries. ( f ) Ratios of apical width to apicobasal length (AW/ABL) in the neural groove cells that are adjacent to midline and express Rab11 constructs (stages 16/17; n , number of examined cells). Means±s.d. are shown on the graph. Rab11-expressing cells are indistinguishable from uninjected control cells (data not shown). ( g ) Rab11 constructs do not affect the neural progenitor fate marker Sox3. ( h ) Medial polarization of GFP-Sec15 in the neural plate of stage 15 embryos. Top view, red rectangle in the inset indicates approximate image position. F-actin marks cell boundaries. ( i – k ) Rab11 polarization depends on planar cell polarity. Immunostaining for endogenous Rab11 in cross-sections of stage 15/16 embryos unilaterally injected with Diversin MO (20 ng, i ), Vangl2 MO (20 ng, j ) or Xdd1 RNA (1 ng, k ). Arrows point to polarized Rab11 on the uninjected side, asterisks indicate lack of Rab11 polarity. Scale bar in j (also refers to i , k ) is 20 μm. M, midline position. GFP-CAAX or GFP RNA (100 pg) served as lineage tracers as indicated. Each result was verified in three to six independent experiments. 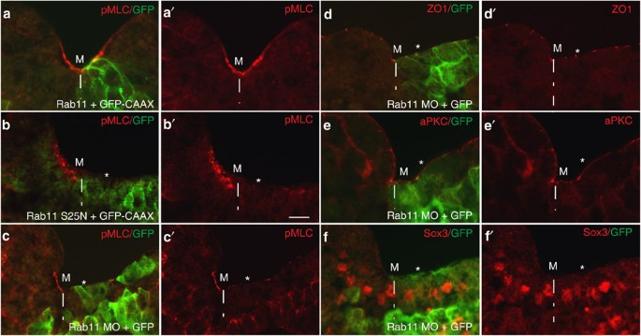Figure 3: Rab11 is required for myosin II activation, but does not affect apicobasal polarity. Four-cell embryos were unilaterally injected with Rab11 (2 ng,a) or Rab11S25N RNA (1 ng,b) or Rab11 morpholino antisense oligonucleotide (MO;c–f), and cultured until neurula stages. Transverse cryosections of the neural groove (stage 17-18) are shown. Asterisk indicates the injected right side, marked by the lineage tracer GFP-CAAX RNA (50 pg, green,a,b) or GFP RNA (50 pg, green,c–f). (a–c) Myosin II activation was assessed by phosphorylated Myosin II light chain (pMLC)-specific immunostaining. Rab11S25N (b,b′) and Rab11 MO (c,c′), but not wild-type Rab11 (a,a′), inhibit apical pMLC staining (red), as compared with the uninjected side. No significant effect is observed on ZO1 (d), aPKC (e) and Sox3 (f). Scale bar is 20 μm (a–f). Asterisk indicates lack of apical pMLC. M, midline position. These results are representative from four to seven independent experiments. Full size image Figure 3: Rab11 is required for myosin II activation, but does not affect apicobasal polarity. Four-cell embryos were unilaterally injected with Rab11 (2 ng, a ) or Rab11S25N RNA (1 ng, b ) or Rab11 morpholino antisense oligonucleotide (MO; c – f ), and cultured until neurula stages. Transverse cryosections of the neural groove (stage 17-18) are shown. Asterisk indicates the injected right side, marked by the lineage tracer GFP-CAAX RNA (50 pg, green, a , b ) or GFP RNA (50 pg, green, c – f ). ( a – c ) Myosin II activation was assessed by phosphorylated Myosin II light chain (pMLC)-specific immunostaining. Rab11S25N ( b , b ′) and Rab11 MO ( c , c ′), but not wild-type Rab11 ( a , a ′), inhibit apical pMLC staining (red), as compared with the uninjected side. No significant effect is observed on ZO1 ( d ), aPKC ( e ) and Sox3 ( f ). Scale bar is 20 μm ( a – f ). Asterisk indicates lack of apical pMLC. M, midline position. These results are representative from four to seven independent experiments. Full size image PCP proteins regulate Rab11 localization in the neural plate Given the medial polarization of Diversin in the neural plate, we hypothesized that PCP signalling could function upstream of Rab11 in neural plate closure. Indeed, neural tube closure defects were apparent in Diversin-depleted embryos ( Supplementary Fig. 3 ). Moreover, interference with the function of Diversin and two other core PCP proteins, Vangl2 and Dishevelled, inhibited Rab11 polarization in the neural plate ( Fig. 2i–k , Supplementary Fig. 4a ). In these experiments, the total amount of Rab11 protein remained unaffected ( Fig. 4a ). Despite the major changes in neural plate morphology and the decrease of myosin II phosphorylation in Vangl2-depleted embryos ( Supplementary Fig. 4b ), Vangl2 MO did not alter the fate of neural progenitors, which remained positive for Sox3 ( Supplementary Fig. 4a ). Finally, coinjection of RNAs encoding Rab11S25N and Vangl2 strongly enhanced the neural tube closure defects observed in separate RNA injections, indicating that these molecules functionally interact ( Supplementary Fig. 4c,d ). These experiments indicate that the polarization of Rab11 endosomes along the mediolateral axis of the neural plate is controlled by the PCP pathway. 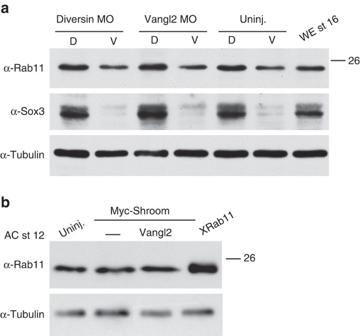Figure 4: Rab11 protein levels in ectodermal cells with manipulated planar cell polarity (PCP) signalling. Embryos were animally injected with Vangl2 morpholino antisense oligonucleotide (MO; 20 ng) or Diversin MO (30 ng) (a) or Rab11 (100 pg), Shroom (0.3 ng) and Vangl2 (1 ng) RNAs (b) and the levels of Rab11 in isolated neural (dorsal, D) and non-neural (ventral, V) explants (stage 16,a) or ectoderm explants made at stage 12 (b) were determined by immunoblot analysis. WE, whole embryo. α-Tubulin is a loading control. The quality of dissection for neural and non-neural explants was assessed by the pan-neural marker Sox3. (a) Although Rab11 levels are higher in neuroectoderm, there was no change after Diversin and Vangl2 depletion. (b) Rab11 levels were not affected in ectoderm explants after Shroom and/or Vangl2 RNA injection; Uninj., uninjected. Figure 4: Rab11 protein levels in ectodermal cells with manipulated planar cell polarity (PCP) signalling. Embryos were animally injected with Vangl2 morpholino antisense oligonucleotide (MO; 20 ng) or Diversin MO (30 ng) ( a ) or Rab11 (100 pg), Shroom (0.3 ng) and Vangl2 (1 ng) RNAs ( b ) and the levels of Rab11 in isolated neural (dorsal, D) and non-neural (ventral, V) explants (stage 16, a ) or ectoderm explants made at stage 12 ( b ) were determined by immunoblot analysis. WE, whole embryo. α-Tubulin is a loading control. The quality of dissection for neural and non-neural explants was assessed by the pan-neural marker Sox3. ( a ) Although Rab11 levels are higher in neuroectoderm, there was no change after Diversin and Vangl2 depletion. ( b ) Rab11 levels were not affected in ectoderm explants after Shroom and/or Vangl2 RNA injection; Uninj., uninjected. Full size image Rab11 functions during ectopic apical constriction As neural plate folding is largely driven by apical constriction of neuroepithelial cells, we suspected that Rab11 has a role in this process. We wanted to examine an alternative model, in which morphogenesis can be separated from neural induction and patterning that accompany neural tube closure. Ectopic apical constriction is induced in blastula ectoderm by overexpression of Shroom, a protein linked to actomyosin contractility and essential for neural tube closure [10] , [28] . We first assessed Rab11 localization during Shroom-induced apical constriction, which took place in the majority of injected embryos ( Fig. 5 ). We observed strong apical recruitment of both Rab11 and Vangl2 in the constricting Shroom-expressing cells, which are easily identified by abundant pigment granules near their apical surfaces and elongated morphology ( Fig. 5a–e , Supplementary Fig. 5a–c ). Moreover, both endogenous and exogenous Rab11 polarized towards the site of Shroom RNA injection in the cells adjacent to the Shroom-expressing tissue ( Fig. 5f–i , Supplementary Fig. 5a,b,e ). Therefore, our lineage tracing analysis suggests that a Shroom-induced signal triggers non-cell-autonomous Rab11 polarization in the surrounding cells. Although it is currently unclear whether Rab11 has the same function in Shroom-expressing and nonexpressing cells, Shroom-dependent apical constriction was inhibited by Rab11S25N in more than 80% of injected embryos ( n =92; Fig. 5j ). Consistent with this morphological effect, Rab11S25N inhibited apical pMLC accumulation induced by Shroom, but had no significant effect on aPKC or ZO1 ( Supplementary Fig. 5h,i , and data not shown). Of interest, overexpressed Vangl2 interfered with Shroom-induced constriction and inhibited Rab11 apical accumulation and planar polarization in Shroom-expressing ectoderm and during neural tube closure ( Supplementary Fig. 5c–g,j,k ), although total Rab11 protein levels in Vangl2-expressing cells did not change ( Fig. 4b ). This Rab11 polarization in cells that respond to Shroom was inhibited by Vangl2 both in the cell autonomous and non-cell autonomous manner ( Supplementary Fig. 5c–g ). Together, these results are consistent with the possibility that the PCP pathway interacts with vesicular trafficking machinery to drive ectopic apical constriction in response to Shroom. 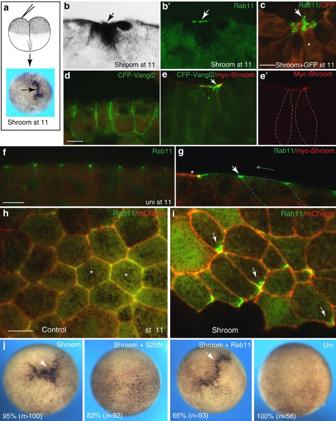Figure 5: Role and localization of Rab11 during ectopic Shroom-induced apical constriction. (a) Scheme of experiments. (b,c) Apical recruitment of Rab11 in response to microinjected Shroom RNA (300 pg). (b) Brightfield image showing pigment accumulation in a constricted cell (arrow). (b′) Anti-Rab11 antibody apical staining of embryo cryosection (arrow). (c)En faceview of apical Rab11 in Shroom-positive cells. GFP RNA is a lineage tracer (red). Arrow points to the constricted apical surface, asterisk indicates cell body. (d,e) Localization of CFP-Vangl2 in stage 11 control ectoderm (d) and at the site of Shroom RNA injection (e,e′). Co-localization of CFP-Vangl2 and myc-Shroom (arrowhead). (f,g) Rab11 polarity in the cells adjacent to Shroom-containing cells. (f) Junctional Rab11 staining in control ectoderm. (g) Rab11 localization (arrow) in cells adjacent to a Shroom-expressing cell (asterisk). Green arrow indicates Rab11 planar polarity, cell boundary is demarcated by dashed line. (h,i) GFP-Rab11 (100 pg) and Shroom (300 pg) RNAs were injected into adjacent blastomeres. Membrane-targeted Cherry RNA (400 pg) was co-injected with GFP-Rab11 RNA to mark cell boundaries. (h) GFP-Rab11 is uniformly present at cell borders in control ectoderm (asterisks). (i) Arrows point to Rab11 polarized towards Shroom-expressing ectoderm (strongly pigmented area at the bottom). Top view is shown, scale bar, 20 μm. (j) Requirement of Rab11 for Shroom-induced constriction. Shroom RNA (300 pg) was coinjected with wild-type Rab11 or Rab11S25N RNA (1 ng each) animally, into four-cell embryos as indicated. Representative embryos are shown at stage 10, numbers indicate percentage of embryos with depicted phenotype. Apical constriction area is heavily pigmented (arrowheads). Figure 5: Role and localization of Rab11 during ectopic Shroom-induced apical constriction. ( a ) Scheme of experiments. ( b , c ) Apical recruitment of Rab11 in response to microinjected Shroom RNA (300 pg). ( b ) Brightfield image showing pigment accumulation in a constricted cell (arrow). ( b ′) Anti-Rab11 antibody apical staining of embryo cryosection (arrow). ( c ) En face view of apical Rab11 in Shroom-positive cells. GFP RNA is a lineage tracer (red). Arrow points to the constricted apical surface, asterisk indicates cell body. ( d , e ) Localization of CFP-Vangl2 in stage 11 control ectoderm ( d ) and at the site of Shroom RNA injection ( e , e ′). Co-localization of CFP-Vangl2 and myc-Shroom (arrowhead). ( f , g ) Rab11 polarity in the cells adjacent to Shroom-containing cells. ( f ) Junctional Rab11 staining in control ectoderm. ( g ) Rab11 localization (arrow) in cells adjacent to a Shroom-expressing cell (asterisk). Green arrow indicates Rab11 planar polarity, cell boundary is demarcated by dashed line. ( h , i ) GFP-Rab11 (100 pg) and Shroom (300 pg) RNAs were injected into adjacent blastomeres. Membrane-targeted Cherry RNA (400 pg) was co-injected with GFP-Rab11 RNA to mark cell boundaries. ( h ) GFP-Rab11 is uniformly present at cell borders in control ectoderm (asterisks). ( i ) Arrows point to Rab11 polarized towards Shroom-expressing ectoderm (strongly pigmented area at the bottom). Top view is shown, scale bar, 20 μm. ( j ) Requirement of Rab11 for Shroom-induced constriction. Shroom RNA (300 pg) was coinjected with wild-type Rab11 or Rab11S25N RNA (1 ng each) animally, into four-cell embryos as indicated. Representative embryos are shown at stage 10, numbers indicate percentage of embryos with depicted phenotype. Apical constriction area is heavily pigmented (arrowheads). Full size image Rab11 and PCP proteins in embryonic wound healing Coordinated changes in cell shape that are similar to apical constriction take place during embryonic wound repair [10] . We further addressed Rab11 function in morphogenesis, by removing a small piece of tissue from blastula ectoderm, a tissue lacking detectable planar polarity ( Fig. 6a ). In this model, wound healing is initiated within minutes after the surgery with pigmented superficial ectoderm spreading eventually over the inner cell layer. Planar polarization of Rab11 became apparent in the superficial layer of the healing tissue in both embryos and ectoderm explants in 30–60 min after the wound was inflicted ( Fig. 6a–c and Supplementary Fig. 6a,b ). We found that both endogenous and exogenous Rab11-containing recycling endosomes are polarized in individual cells towards the direction of the wound ( Fig. 6a–e , Supplementary Fig. 6a,b ). In addition, both Rab11 and Vangl2 protein complexes became apically enriched in inner ectoderm cells, which are known to participate in apical constriction during wound closure [10] ( Supplementary Fig. 6b , asterisk, Supplementary Fig. 7 ). Moreover, wound healing was defective in embryos and explants that expressed Rab11S25N, Rab11 MO or Vangl2 MO ( Fig. 6f–h , Supplementary Fig. 6c–i ), indicating that both Rab11 and Vangl2 are required for this process. Similar to our observations of neural plate folding, Vangl2 depletion inhibited Rab11 polarization and pMLC accumulation (data not shown). Cumulatively, our findings suggest that polarized Rab11-mediated recycling is involved in diverse models of epithelial morphogenesis and point to the conservation of mechanisms regulating neural tube closure and embryonic wound healing. 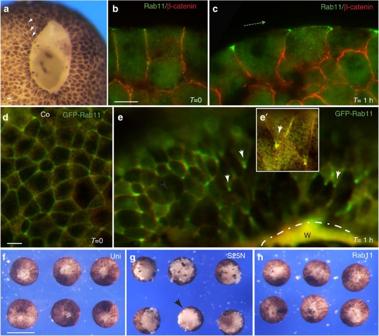Figure 6: Planar polarity of Rab11 endosomes during epithelial wound healing. (a) Representative blastula embryo (stage 9), 30 min after wounding. Arrowheads point to polarized cells. (b) Rab11 staining in control ectoderm. (c) Representative ectodermal explant with Rab11 polarization relative to the wound position. Costaining with β-catenin antibodies indicates cell boundaries. Dashed green arrow indicates the direction towards the wound. (d,e) Live images of GFP-Rab11 polarization (white arrows) in ectoderm during wound healing. (d) Control ectoderm; (e) explant with wound healing for 1 h. Wound (W) position is indicated by broken line. (e′) Inset shows two individual cells with polarized GFP-Rab11. (f–h) Rab11 is essential for wound healing in ectodermal explants. Ectodermal explants were prepared at late blastula stages from the uninjected embryos (f), or embryos injected with wild-type Rab11 (h) or Rab11S25N (g) RNAs (1 ng each), and allowed to heal for 1 h at room temperature. Scale bars are 20 μm inbandd, also refer toc,e, and 300 μm inf, also refers tog,h. Results are representative of three to five independent experiments. Figure 6: Planar polarity of Rab11 endosomes during epithelial wound healing. ( a ) Representative blastula embryo (stage 9), 30 min after wounding. Arrowheads point to polarized cells. ( b ) Rab11 staining in control ectoderm. ( c ) Representative ectodermal explant with Rab11 polarization relative to the wound position. Costaining with β-catenin antibodies indicates cell boundaries. Dashed green arrow indicates the direction towards the wound. ( d , e ) Live images of GFP-Rab11 polarization (white arrows) in ectoderm during wound healing. ( d ) Control ectoderm; ( e ) explant with wound healing for 1 h. Wound (W) position is indicated by broken line. ( e′ ) Inset shows two individual cells with polarized GFP-Rab11. ( f – h ) Rab11 is essential for wound healing in ectodermal explants. Ectodermal explants were prepared at late blastula stages from the uninjected embryos ( f ), or embryos injected with wild-type Rab11 ( h ) or Rab11S25N ( g ) RNAs (1 ng each), and allowed to heal for 1 h at room temperature. Scale bars are 20 μm in b and d , also refer to c , e , and 300 μm in f , also refers to g , h . Results are representative of three to five independent experiments. Full size image Several models of epithelial folding have been proposed including coordinated regulation of actomyosin contractility [2] , [3] , [6] , [9] , repositioning of adherens junctions by PAR proteins [5] and enhanced endocytosis [20] . Despite the recent progress, it remained unclear whether tissue folding has any directionality. Our experiments visualizing the graded distribution of Rab11 recycling endosomes are the first to reveal the cell polarity corresponding to the axis of bending or constriction. We also find that this polarity requires core PCP proteins, reinforcing the known connection between vesicular trafficking and PCP [19] , [29] , [30] , [31] , [32] . The unique localization of Rab11 and the exocyst component Sec15 suggests a model with an essential role of anisotropic membrane trafficking in neural tube closure. In this model, PCP signals are conveyed to individual cells to polarize Rab11-mediated membrane trafficking and allow apical constriction to proceed directionally, towards the midline, by expanding the lateral membrane domain at the expense of the shrinking apical domain. Although our experiments demonstrate a requirement of Rab11 for myosin II activation in the neural plate, we note that the proposed mechanism does not support the classical ‘purse string’ model with isotropic actomyosin contractility along the mediolateral axis. The same general mechanism may act to polarize membrane trafficking in individual cells in response to wounding, leading to cell reorientation and tissue repair. The observed regulation of Rab11-dependent vesicular trafficking by core PCP molecules reiterates novel roles of these proteins in modulating cell shape and behaviour during tissue folding and embryonic wound healing. Nevertheless, Rab11 roles in cell elongation, radial intercalation or convergent extension during neural tube closure [1] , and relevant cargo proteins for Rab11 vesicles remain to be elucidated. Consistent with the possibility that Vangl2 trafficking depends on Rab11, CFP-Vangl2 membrane localization became more diffuse and shifted to the cytoplasm in cells depleted of Rab11 or expressing Rab11S25N ( Supplementary Fig. 8 ). This finding supports a positive feedback loop, in which PCP proteins that regulate Rab11 are themselves targeted to their specific locations by Rab11-dependent trafficking [31] , [33] , [34] . Plasmids, microinjections, in situ hybridization Plasmids encoding GFP-C1, GFP-Rab11, GFP-Rab11S25N in pXT7, untagged Rab11, Rab11S25N, Rab11Q70L in pXT7 and GFP-CAAX in pCS2 (ref. 23 ); mouse Shroom/ShrmL (also known as Shroom3) [28] and Xdd1-pCS2 (ref. 35 ) have been previously described. Whole-mount in situ hybridization and Xgal staining were carried out using standard techniques [36] with the digoxigenin-labelled antisense probes for Nrp1 (ref. 37 ) and Rx1 (ref. 38 ). Myc-Shroom in pCS2+ was generated by subcloning of Shroom/ShrmL. For lineage tracing, GFP or membrane-targeted GFP-CAAX (50–100 pg) or membrane-targeted mCherry (400 pg) RNA was injected along with morpholino antisense oligonucleotides (MOs) or RNAs. Capped mRNA was made by in vitro transcription with T7 or SP6 promoter using mMessage mMachine kit (Ambion). Rab11 MO [23] , control MO [23] , Vangl2/Stbm MO [39] and Diversin MO [40] and the constructs for HA-Diversin-RFP in pCS105, CFP-Vangl2 (Stbm) [41] and rat Myc-GFP-Sec15 (ref. 42 ) have been described. The Pk plasmid was a gift from Jenny. Myc-GFP-Sec15 was subcloned into pXT7 vector. Details of cloning are available upon request. Xenopus embryo injections, apical constriction and wound-healing assays In vitro fertilization, culture and staging of Xenopus laevis embryos were carried out following standard techniques [23] . This study was carried out in strict accordance with the recommendations of the Guide for the Care and Use of Laboratory Animals of the National Institutes of Health. The protocol 04–1295 was approved by the Institutional Animal Care and Use Committee of the Icahn School of Medicine at Mount Sinai. For microinjections, four-cell embryos were transferred into 2% Ficoll in 0.3 × MMR buffer [43] and 5–10 nl of mRNAs or MO solution was injected into one or more blastomeres. Amounts of injected mRNA or MO per embryo have been optimized in preliminary dose-response experiments (data not shown) and are indicated in figure legends. For ectopic apical constriction, 4- to 8-cell embryos were injected animally into one dorsal and one ventral animal blastomere. Wound healing was modelled by removing a small piece of animal pole ectoderm from Xenopus blastulae at stages 9–9.5. Embryos and explants were cultured in 0.7 × MMR solution for 30–60 min, and were imaged live or fixed for cryosections. Embryonic defects were scored as the percentage of embryos with the representative phenotype, based on several independent experiments. Experimental groups contained 25–35 embryos per group, and each result was verified in three to six independent experiments. Immunohistochemistry and immunoblot analysis To examine protein subcellular localization, neural plate explants expressing GFP- or RFP-tagged constructs were dissected at stages 15–17 from embryos fixed for 1 h with MEMFA (0.1 M 3-( N -Morpholino)-propanesulfonic acid, pH 7.4, 2 mM EGTA, 1 mM MgSO 4 and 3.7% formaldehyde), washed with 1 × PBS and mounted for observation with the Vectashield mounting medium (Vector). Ectoderm explants expressing GFP-tagged constructs were dissected at stage 11 and processed as described above. For F-actin staining, Alexa 568-conjugated phalloidin (5 U ml −1 , Molecular Probes) was used. For detection of Rab11 and pMLC on cryosections, embryos were devitellinized, fixed with 2% trichloracetic acid solution for 30 min at room temperature and washed with 0.3% Triton X-100 in 1 × PBS for 30 min (ref. 44 ). For en face view of Rab11 and ZO1 in the neural plate, explants were fixed with trichloracetic acid [44] and stained with primary antibodies overnight, secondary antibody for 2 h, washed and mounted for imaging. Cryosectioning and immunostaining were performed as described in Dollar et al. [43] Briefly, the embryos were embedded in the solution containing 15% cold fish gelatin and 15% sucrose, sectioned at 10 μm and immunostained overnight. Antibodies against the following antigens were used: Rab11 (1:50-100, Invitrogen, rabbit polyclonal and rabbit monoclonal, and 1:100, BD Biosciences), GFP (1:200, B-2, mouse monoclonal, Santa Cruz or rabbit polyclonal, Invitrogen), ZO-1 (1:200, mouse, Invitrogen; rabbit, Zymed), PKCζ (1:200, C-20, rabbit polyclonal, Santa Cruz), Sox3 (1:200, rabbit polyclonal, a gift of Klymkowsky), β-catenin (1:200, rabbit polyclonal, Sigma), pMLC (anti-phospho-Ser20 myosin light chain; 1:300; rabbit polyclonal, Abcam), anti-myc (1:60, 9E10 hybridoma supernatant). Secondary antibodies were against mouse or rabbit IgG conjugated to Alexa Fluor-488, Alexa Fluor-555 (1:100, Invitrogen) or Cy3 (1:100, Jackson ImmunoResearch). Cryosections were mounted for observation with the Vectashield mounting medium (Vector). Standard specificity controls were performed to confirm lack of cross-reactivity and no staining without primary antibodies. Cell shape was assessed as the ratio of apical width to apicobasal length in the neural groove cells next to midline. Immunofluorescence images were captured using the Axioimager fluorescence microscope (Zeiss) and Axiovision imaging software (Zeiss). Results are shown as representative images from at least three independent experiments, each containing 10–20 embryos per group. Fluorescent projection images were obtained with a Leica SP5 confocal microscope (Leica). Immunoblot analysis was done with dissected tissues (neural plate explants, stage 16, or animal caps, stage 12) with anti-Rab11, anti-Sox3 and anti-α−tubulin antibodies using standard techniques [45] . Briefly, embryos were resuspended in lysis buffer (0.5% Triton X-100, 10 mM Tris–HCI at pH 7.5, 50 mM NaCl, 1 mM EDTA), containing protease inhibitor cocktail (Roche). Proteins were resolved by SDS–polyacrylamide gel electrophoresis. An equivalent of 0.2–0.5 embryo was loaded per lane. After protein transfer to the Immobilon-P PVDF membrane (Millipore), the membrane was incubated sequentially with primary and secondary antibodies, conjugated to horseradish peroxidase. Peroxidase activity was detected by enhanced chemiluminescence. How to cite this article: Ossipova, O. et al. Role of Rab11 in planar cell polarity and apical constriction during vertebrate neural tube closure. Nat. Commun. 5:3734 doi: 10.1038/ncomms4734 (2014).